Quantitative live-cell imaging reveals spatio-temporal dynamics and cytoplasmic assembly of the 26S proteasome The 26S proteasome is a 2.5-MDa multisubunit protease complex that degrades polyubiquitylated proteins. Although its functions and structure have been extensively characterized, little is known about its dynamics in living cells. Here, we investigate the absolute concentration, spatio-temporal dynamics and complex formation of the proteasome in living cells using fluorescence correlation spectroscopy. We find that the 26S proteasome complex is highly mobile, and that almost all proteasome subunits throughout the cell are stably incorporated into 26S proteasomes. The interaction between 19S and 20S particles is stable even in an importin-α mutant, suggesting that the 26S proteasome is assembled in the cytoplasm. Furthermore, a genetically stabilized 26S proteasome mutant is able to enter the nucleus. These results suggest that the 26S proteasome completes its assembly process in the cytoplasm and translocates into the nucleus through the nuclear pore complex as a holoenzyme. The 26S proteasome is a multisubunit protease that degrades polyubiquitinated proteins in an ATP-dependent manner [1] , [2] , [3] . It is involved in a wide variety of cellular processes, and proteasomal dysfunctions lead to a variety of diseases [4] . The 26S proteasome is composed of at least 33 different subunits, organized into two particles: a highly conserved 20S core particle (CP), containing the central catalytic cavity, and one or two 19S regulatory particles (RPs). The CP is a barrel-shaped structure of ~730 kDa, consisting of four heptameric rings, whereas the RP is a ~930-kDa complex consisting of 19 different subunits. The RP mediates multiple aspects of proteasome function such as recognition, deubiquitylation and unfolding of substrates and translocation of substrates into the CP. The RP can be separated into two major subcomplexes, the base and the lid [3] . The base includes six different AAA+ATPase subunits (Rpt1–6) and three non-ATPase subunits (Rpn1, 2 and 13), whereas the lid consists of nine non-ATPase subunits (Rpn3, 5–9, 11, 12 and 15). The lid partially surrounds the ATPase ring of the base, and two ubiquitin receptors, Rpn10 and Rpn13, are located on the periphery of the 19S RP [5] , [6] , [7] , [8] . Recent studies have suggested that the assembly of the proteasome proceeds via a highly ordered multistep mechanism [9] , [10] , [11] , [12] . All of the subcomplexes of the proteasome (CP, base, and lid) seem to assemble independently; the CP and base require multiple proteasome-dedicated chaperones for efficient and correct assembly. In proliferating yeast and some cultured mammalian cells, the 26S proteasome is highly enriched in the nucleus, where it is involved in degradation of nuclear proteins [13] , [14] , [15] , [16] , [17] . Because only a small number of proteasome subunits contain a nuclear localization signal (NLS) [13] , [18] , [19] , and because yeast undergoes a closed mitosis in which the nuclear envelope remains intact and mitosis occurs within the nucleus, the yeast proteasome must enter the nucleus in an at least partially assembled form. In support of this notion, previous studies have shown that CP components are imported into the nucleus as inactive precursor complexes via the importin-α/β pathway [20] . Additional evidence suggests that the CP and the lid and base subcomplexes are imported separately [19] , [21] . These observations imply that the yeast 26S proteasome is assembled inside the nucleus from independently imported modules. By contrast, other studies have suggested that the holoenzyme or novel form of the preassembled proteasome undergoes nuclear translocation [22] , [23] , [24] . Because the channel of the nuclear pore complex (NPC) can expand to accommodate cargoes with a diameter of up to 39 nm, as revealed by studies using gold particles [25] , it is theoretically possible for intact CP or even the entire 26S proteasome to pass through the NPC. However, the inner channel of the NPC is largely composed of unstructured FG-repeat-containing nucleoporins that create a hydrophobic meshwork that acts as a permeability barrier [26] , potentially preventing the translocation of the proteasome. Therefore, it remains unclear whether the intact 26S proteasome can pass through the NPC. In this study, we investigated the absolute concentration, dynamics, and complex formation of the 26S proteasome in living yeast cells by fluorescence correlation spectroscopy (FCS) [27] , [28] , [29] , [30] , a method for quantitative live-cell imaging. Unexpectedly, we found that the 26S proteasome is a highly mobile complex, and that almost all proteasome subunits are stably incorporated into 26S proteasomes in both the cytosol and nucleus. Complex formation is not significantly altered in an importin-α mutant, suggesting that the proteasome is assembled in the cytosol. Consistent with this, a genetically stabilized 26S proteasome in which the RP and CP are fused does not exhibit any obvious defects and is distributed normally in the nucleus. These results suggest that the 26S proteasome can complete its assembly process in the cytoplasm and translocate into the nucleus through the NPC as a holoenzyme. Dynamics of the 26S proteasome revealed by FCS FCS [27] , [28] , [29] measures fluorescence fluctuations within a defined volume, determined by the laser and the optical setup, to determine a correlation function for probe molecules ( Fig. 1 ). Fitting of mathematical models of the fluorescence correlation function (FCF) allows determination of the concentration of the target complex, as well as its the diffusion coefficient ( D ), which is directly related to molecular weight and shape ( Fig. 1 ). We first investigated whether these methods could be applied to macromolecules in extracts from cells expressing chromosomally green fluorescent protein (GFP)-tagged proteasome subunit (Pre6) [14] , [21] , Hsp104, or ribosome subunit Rpl19a ( Fig. 2 ) [31] , [32] , [33] . All of the FCF curves fit well to a one-component diffusion model ( Fig. 2 ), suggesting that each of these macromolecules were present as a single entity in the extract. 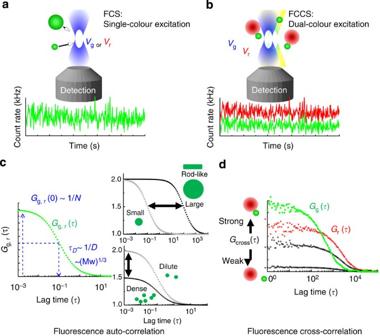Figure 1: Schematic diagram for FCS and FCCS setup and parameters. (a) One-color fluorescence auto-correlation (FCS) and (b) dual-color cross-correlation spectroscopy (FCCS) are methods based on fluctuation analysis of fluorescence intensity (count rate or c.p.s., kHz) detected from a tiny open volume (VgorVrfor FCS,VgandVrfor FCCS). Subscripts g and r represent green and red fluorescent probes, respectively. (c) FCS provides a fluorescence auto-correlation function (GgorGr), allowing measurement of two important biophysical parameters: the average number of fluorescent molecules (N) in a detection volume and the translational diffusion time (τD) of the molecules through the open volume. Mobility parameter (τDorD) of molecules reflects the molecular size (MW orRh), shape of fluorescent species, and the apparent viscosity in solution or in a live cell (see also Methods). (d) Dual-color FCCS provides a cross-correlation function (Gcross, represented byGcin the main text) and two auto-correlation functions (GgandGr), respectively.Gcallows measurement of direct interaction or colocalization of a green and red fluorescent molecules transiting through open volumesVgandVr, in addition to the parameters for one-color FCS as described inc. The molecular weights (MW fcs ) estimated from the measured D values for Hsp104 and the proteasome were larger than their theoretical molecular weights ( Table 1 ). However, this inconsistency can be explained by a model using standard spherical particles ( Supplementary Fig. 1a ) that takes into account the shapes of Hsp104 and the proteasome, including the presence of cavities in these complexes ( Supplementary Fig. 1b–d ). Figure 1: Schematic diagram for FCS and FCCS setup and parameters. ( a ) One-color fluorescence auto-correlation (FCS) and ( b ) dual-color cross-correlation spectroscopy (FCCS) are methods based on fluctuation analysis of fluorescence intensity (count rate or c.p.s., kHz) detected from a tiny open volume ( V g or V r for FCS, V g and V r for FCCS). Subscripts g and r represent green and red fluorescent probes, respectively. ( c ) FCS provides a fluorescence auto-correlation function ( G g or G r ), allowing measurement of two important biophysical parameters: the average number of fluorescent molecules ( N ) in a detection volume and the translational diffusion time ( τ D ) of the molecules through the open volume. Mobility parameter ( τ D or D ) of molecules reflects the molecular size (MW or R h ), shape of fluorescent species, and the apparent viscosity in solution or in a live cell (see also Method s ). ( d ) Dual-color FCCS provides a cross-correlation function ( G cross , represented by G c in the main text) and two auto-correlation functions ( G g and G r ), respectively. G c allows measurement of direct interaction or colocalization of a green and red fluorescent molecules transiting through open volumes V g and V r , in addition to the parameters for one-color FCS as described in c . 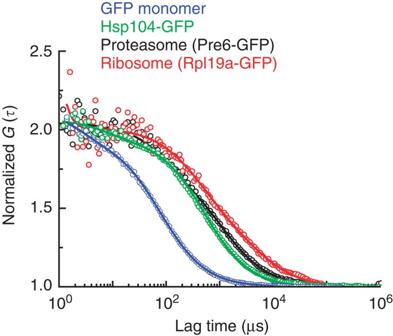Figure 2: Quantitation by FCS of GFP-tagged macromolecules in extracts. FCS analysis of the proteasome and giant protein complexes in yeast lysates. Extracts from cells expressing monomeric GFP (YCP001), Hsp104-GFP (YCP003), Pre6-GFP (YYS1033) or Rpl19a-GFP (YCP004) were analysed by FCS. Representative normalized FCF curves of different sizes of proteins are shown (circle symbol). For comparison of mobility, all of the curves were normalized to the same amplitude,G(0)=2. Solid lines indicate fitting of one-component models to the results. Full size image Figure 2: Quantitation by FCS of GFP-tagged macromolecules in extracts. FCS analysis of the proteasome and giant protein complexes in yeast lysates. Extracts from cells expressing monomeric GFP (YCP001), Hsp104-GFP (YCP003), Pre6-GFP (YYS1033) or Rpl19a-GFP (YCP004) were analysed by FCS. Representative normalized FCF curves of different sizes of proteins are shown (circle symbol). For comparison of mobility, all of the curves were normalized to the same amplitude, G (0)=2. Solid lines indicate fitting of one-component models to the results. Full size image Table 1 Summary of calculated molecular weights (MW) and diffusion coefficients ( D ) of GFP-tagged macromolecules in extracts. Full size table We next applied FCS to living yeast cells ( Fig. 3 ; Supplementary Fig. 2 ). To elucidate the dynamics of all subcomplexes of the proteasome at their endogenous expression levels, we studied yeast cells expressing chromosomally GFP-tagged Pre6 (a CP subunit), Rpn1 (a base subunit) or Rpn7 (a lid subunit) ( Fig. 3a ). Exponentially growing cells were mounted on a glass-bottom dish to eliminate possible mechanical stress [34] . We measured proteasome dynamics in both the cytoplasm and nucleus. The FCF curves in both compartments were very similar for all three subunits ( Fig. 3b ; Supplementary Fig. 3 ). Unexpectedly, the mobilities of the subunits in live cells had two or more components, rather than the simple one-component diffusion observed in extracts. Because a two-component diffusional model fitted well to the FCF curves (see Methods), we conclude that almost all proteasome subunits exist within cells as components of two species. Based on our previous finding that the apparent viscosity in the yeast cell is ~4 cP (ref. 31 ), we calculated that the size of one of these species (represented by D fast ) is 1–10 MDa, whereas the size of the other (represented by D slow ) is ~32 GDa ( Table 2 ). The smaller species seemed to represent the bona fide 26S proteasome ( Supplementary Fig. 4 ), whereas the larger species seemed to represent a novel form of the proteasome, possibly reflecting strong interactions with other cellular components. From the initial amplitude of the correlation curve, G (0), we calculated the absolute concentrations of the proteasome subunits: 140–200 nM in the cytoplasm and 830–980 nM in the nucleus ( Fig. 3c ). 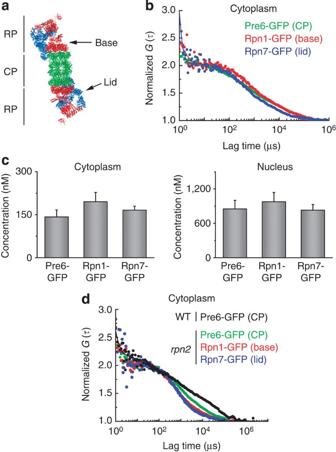Figure 3: Quantitation by FCS of GFP-tagged proteasome subunits in living cells. (a) The structure of the 26S proteasome adapted the atomic structural model (PDB ID: 4B4T). Subcomplexes of the proteasome are indicated: CP in green, base in red and lid in blue. (b) FCS analysis of proteasome subunits in living yeast cells. Normalized FCF curves are shown for Pre6-GFP (CP, YYS1033), Rpn1-GFP (base, YYS1034) and Rpn7-GFP (lid, YYS1035), measured in the cytoplasm. Solid lines indicate fitting of two-component models to the results. See Methods in detail. (c) Absolute concentrations of proteasome subunits in the cytoplasm and nucleus. The concentrations of proteasome subunits in living cells were calculated from measured FCFs (means±s.e.m.;n=45 cells). (d) FCS analysis of proteasome subunits inrpn2mutant cells.rpn2mutant cells expressing Pre6-GFP (CP, YYS2110), Rpn1-GFP (base, YYS2111), or Rpn7-GFP (lid, YYS2112) were analysed by FCS. Normalized FCF curves measured in the cytoplasm are shown. For comparison of mobility, all of the curves inbanddwere normalized to the same amplitude,G(0)=2. Solid lines indicate fitting of two-component model to the results. Figure 3: Quantitation by FCS of GFP-tagged proteasome subunits in living cells. ( a ) The structure of the 26S proteasome adapted the atomic structural model (PDB ID: 4B4T). Subcomplexes of the proteasome are indicated: CP in green, base in red and lid in blue. ( b ) FCS analysis of proteasome subunits in living yeast cells. Normalized FCF curves are shown for Pre6-GFP (CP, YYS1033), Rpn1-GFP (base, YYS1034) and Rpn7-GFP (lid, YYS1035), measured in the cytoplasm. Solid lines indicate fitting of two-component models to the results. See Methods in detail. ( c ) Absolute concentrations of proteasome subunits in the cytoplasm and nucleus. The concentrations of proteasome subunits in living cells were calculated from measured FCFs (means±s.e.m. ; n =45 cells). ( d ) FCS analysis of proteasome subunits in rpn2 mutant cells. rpn2 mutant cells expressing Pre6-GFP (CP, YYS2110), Rpn1-GFP (base, YYS2111), or Rpn7-GFP (lid, YYS2112) were analysed by FCS. Normalized FCF curves measured in the cytoplasm are shown. For comparison of mobility, all of the curves in b and d were normalized to the same amplitude, G (0)=2. Solid lines indicate fitting of two-component model to the results. Full size image Table 2 Comparisons of the proteasome mobility between wild-type and rpn2 cells. Full size table As a control for our in vivo measurements of proteasome dynamics, we analysed a mutant of Rpn2, the second largest subunit of the proteasome, in which proteasome assembly is defective. In the rpn2 mutant, the 26S proteasome was almost completely disassembled into the lid, base (lacking Rpn2) and CP even at the permissive temperature [21] . Indeed, the FCF curves of Pre6-GFP, Rpn1-GFP and Rpn7-GFP were dramatically altered ( Fig. 3d and Table 2 ). D fast values for Pre6-GFP, Rpn1-GFP and Rpn7-GFP were twofold larger than in wild-type cells, indicating ~8-fold reductions of their MW fcs . This experiment illustrates that dissociation of the holo-proteasome into its constituent subcomplexes can be monitored by FCS analysis, and that FCS analysis can be applied to the in vivo measurement of proteasome dynamics. Next, we sought to characterize the slower-mobility species with an apparent molecular weight of ~32 GDa. We hypothesized that the very slow correlation might reflect binding and unbinding to immobile cellular components. The fractional ratios of D fast and D slow differed slightly between the cytosol and the nucleus, but overall ~40% of total proteasomes in both compartments appeared to be associated with cellular components ( Table 2 ; Supplementary Fig. 3 ). Notably, in rpn2 cells, the fraction of the slower-mobility species decreased to ~20%, suggesting that fully assembled proteasomes, rather than constituent subcomplexes, associate with these cellular components. Recent studies suggested that cytoplasmic proteasomes interact directly with actin fibres [35] , and that nuclear proteasomes associate with chromatin during the transcription process [36] . To test these ideas, we exposed cells to drugs targeting these features of the cell. Disruption of actin fibres by latrunculin A did not affect proteasome mobilities ( Supplementary Fig. 5a,b ), suggesting that the proteasomes do not associate with an intact actin cytoskeleton. By contrast, inhibition of RNA polymerase II by actinomycin D decreased the fraction of the slower-mobility proteasomes ( Supplementary Fig. 5c ), suggesting that a large fraction of proteasomes is engaged with actively transcribed chromatin in the nucleus. Further studies are needed to determine the proteasome-associated cellular components in the cytoplasm. The 26S proteasome is a very stable complex in living cells Dual-color fluorescence cross-correlation spectrometry (FCCS) is designed to examine complex formation between two molecules labelled with different colours (e.g., GFP and mCherry, Fig. 1 ) [27] , [28] , [29] . The observations described above indicated that almost all proteasome subunits exist as the 26S proteasome. To confirm these findings, we carried out FCCS analysis in cells co-expressing Rpn7-GFP (lid) and Pre6-mCherry (CP) ( Fig. 4a ). If the lid subunit and the CP subunit exist in the same complex, we should observe co-diffusion of GFP and mCherry as they enter and leave the focal volume, represented by the amplitude of cross-correlation, G c (0) [27] , [28] , [29] . As shown in Fig. 4b , high cross-correlation was indeed observed between Rpn7-GFP and Pre6-mCherry. The relative interaction amplitude between Rpn7-GFP and Pre6-mCherry, represented by [ G c (0)−1]/[ G g or r (0)−1], was larger than that of a GFP–mCherry fusion protein, suggesting that the RP–CP interaction is quite strong ( Fig. 4c ). Notably, the same result was obtained in both the cytoplasm and nucleus. Thus, FCCS analysis revealed that the 26S proteasome is a very stable complex in live cells. 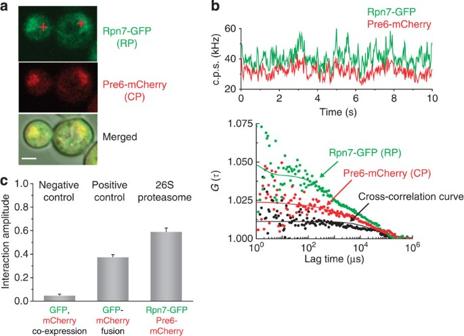Figure 4: Stable complex formation of the 26S proteasome in living cells. (a) Fluorescence-microscopic image ofRPN7-GFP PRE6-mCherrycells (YYS1163). Scale bar, 2 μm. (b) Representative FCCS measurement of theRPN7-GFP PRE6-mCherrycells. (Upper) Change over time of average fluorescence intensity (counts per second; cps in kHz). (Bottom) Two corresponding FCFs (green and red) and one FCCS curve (black) indicate a strong interaction. (c) Summary of interaction amplitude of the RP–CP interaction. Interaction amplitude represents the mean value of the relative cross-correlation amplitude. As controls, cells co-expressing GFP and mCherry protein (negative control, YCP002) or GFP–mCherry fusion protein (positive control, YYS1419) were also analyzed (means±s.e.m.;n=15). Figure 4: Stable complex formation of the 26S proteasome in living cells. ( a ) Fluorescence-microscopic image of RPN7-GFP PRE6-mCherry cells (YYS1163). Scale bar, 2 μm. ( b ) Representative FCCS measurement of the RPN7-GFP PRE6-mCherry cells. (Upper) Change over time of average fluorescence intensity (counts per second; cps in kHz). (Bottom) Two corresponding FCFs (green and red) and one FCCS curve (black) indicate a strong interaction. ( c ) Summary of interaction amplitude of the RP–CP interaction. Interaction amplitude represents the mean value of the relative cross-correlation amplitude. As controls, cells co-expressing GFP and mCherry protein (negative control, YCP002) or GFP–mCherry fusion protein (positive control, YYS1419) were also analyzed (means±s.e.m. ; n =15). Full size image The 26S proteasome can form in the cytoplasm Our FCS analysis did not detect proteasome assembly intermediates in wild-type cells, probably because such intermediates are not abundant [37] , [38] , [39] , [40] . Previous studies using a specific importin-α mutant, srp1-49 , suggested that nucleocytoplasmic transport mediated by importin α/β is coupled to proteasome biogenesis [19] , [20] , [21] , [23] . We hypothesized that proteasome intermediates might be detected in the srp1-49 mutant. To test this idea, we analysed proteasome dynamics in the srp1-49 mutant by FCS/FCCS. As reported previously, when cultures of srp1-49 cells were shifted to the restrictive temperature for 6 h, corresponding to four doubling times, newly synthesized proteasome subunits were retained in the cytoplasm and accumulated at the outer membrane of the nuclear envelope [21] ( Fig. 5a ). Under these conditions, we determined the absolute concentrations of the proteasome subunits. In srp1-49 cells, the concentration of each subunit was increased 2-fold in the cytoplasm relative to the concentration in wild-type cells, whereas the nuclear concentrations were decreased threefold ( Fig. 5b ). Unexpectedly, we did not detect assembly intermediates or free subcomplexes in srp1-49 cells by FCS. This observation raised the possibility that the proteasome is assembled in the cytoplasm. To monitor the assembly status of the proteasome complex, we constructed an srp1-49 RPN7-GFP PRE6-mCherry strain and analysed it by FCCS. The relative cross-correlation amplitudes between Rpn7-GFP and Pre6-mCherry did not change over 3 or 6 h of culture (two or four doublings, respectively) at the restrictive temperature ( Fig. 5c ). Accordingly, the interaction amplitudes changed only slightly in both the cytoplasm and the nucleus ( Fig. 5d ). These results suggest that the 26S proteasome was still able to form in the cytoplasm even when nuclear import is impaired. 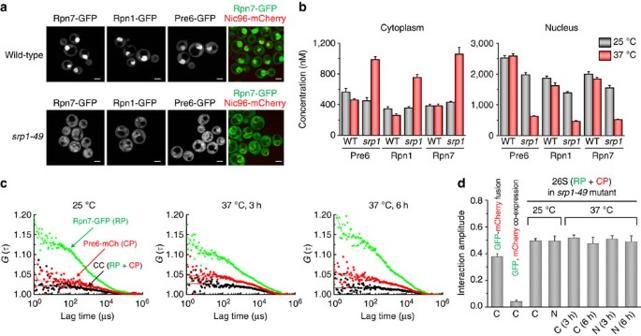Figure 5: FCS and FCCS analyses of the proteasome in an importin-α mutant. (a) Cytoplasmic accumulation of the proteasome subunit in an importin-α mutant. Wild-type or importin-α mutant (srp1-49) cells expressing GFP-tagged proteasome subunits (YSO11, 12, 33, 34, 47 and 52), and cells expressing mCherry-tagged Nic96, a component of the nuclear pore complex (YYS1969 and 1970), were cultured for 6 h at 37 °C (corresponding to four doubling times) and imaged by confocal microscopy. Scale bars, 2 μm. (b) Absolute concentrations of proteasome subunits insrp1-49cells. The concentrations of the proteasome subunits in the cytoplasm and nucleus were determined at both permissive (25 °C) and restrictive (37 °C, 6 h) temperatures (means±s.e.m.;n=15). (c) FCCS measurement ofsrp1-49 RPN7-GFP PRE6-mCherrycells. Representative FCCS curves fromsrp1-49 RPN7-GFP PRE6-mCherrycells (YYS1745) under the indicated conditions. CC, cross-correlation curve. (d) Summary of interaction amplitude of the RP–CP interaction insrp1-49mutant cells. Interaction amplitude, representing the mean value of the relative cross-correlation amplitude, was calculated from the correlation curves measured in live cells under each condition (means±s.e.m.;n=15). Figure 5: FCS and FCCS analyses of the proteasome in an importin-α mutant. ( a ) Cytoplasmic accumulation of the proteasome subunit in an importin-α mutant. Wild-type or importin-α mutant ( srp1-49 ) cells expressing GFP-tagged proteasome subunits (YSO11, 12, 33, 34, 47 and 52), and cells expressing mCherry-tagged Nic96, a component of the nuclear pore complex (YYS1969 and 1970), were cultured for 6 h at 37 °C (corresponding to four doubling times) and imaged by confocal microscopy. Scale bars, 2 μm. ( b ) Absolute concentrations of proteasome subunits in srp1-49 cells. The concentrations of the proteasome subunits in the cytoplasm and nucleus were determined at both permissive (25 °C) and restrictive (37 °C, 6 h) temperatures (means±s.e.m. ; n =15). ( c ) FCCS measurement of srp1-49 RPN7-GFP PRE6-mCherry cells. Representative FCCS curves from srp1-49 RPN7-GFP PRE6-mCherry cells (YYS1745) under the indicated conditions. CC, cross-correlation curve. ( d ) Summary of interaction amplitude of the RP–CP interaction in srp1-49 mutant cells. Interaction amplitude, representing the mean value of the relative cross-correlation amplitude, was calculated from the correlation curves measured in live cells under each condition (means±s.e.m. ; n =15). Full size image To rule out the possibility that cytoplasmic accumulation of the subcomplexes artificially induced formation of 26S proteasomes, we deleted RPN4 from srp1-49 cells. Rpn4 is a transcription factor that regulates proteasome concentrations; deletion of RPN4 significantly reduces the levels of proteasome subunits [39] , [41] . Consistent with this, the cytoplasmic concentration of Rpn7-GFP, measured by FCS, decreased to ~160 nM in srp1-49 rpn4Δ double-mutant cells at both the permissive and non-permissive temperatures ( Supplementary Fig. 6 ). Next, we analysed these cells by FCCS. Although the interaction amplitude between Rpn7-GFP and Pre6-mCherry in the srp1-49 rpn4Δ mutant was slightly lower than that in wild-type cells, it did not change at the non-permissive temperature. Thus, 26S proteasomes could still form in srp1-49 rpn4Δ mutant cells. Together, these results suggest that nuclear import is not required for the formation of the 26S proteasome. Stabilized holoproteasomes are localized in the nucleus Our results obtained from live-cell measurements demonstrate that the 26S proteasome can form in the cytoplasm, and then enter the nucleus. As noted above, the channel of the NPC can expand to 39 nm (ref. 25 ), the 26S proteasome could translocate into the nucleus through via the NPC. However, the inner channel of the NPC serves as a permeability barrier [26] , which potentially prevents translocation of the 26S proteasome as intact complex. The 26S proteasome is intrinsically unstable: it is easily dissociated into the RP and the CP in vitro , and recent studies have also suggested that the RP–CP interface is structurally fragile on exposure to oxidative stress in vivo [42] . Because only a few proteasome subunits contain NLS sequences, dissociation might occur at the subcomplex level, especially at the RP–CP interface. In our FCCS measurements, the time resolution is limited to >10 μs, therefore, the data described above cannot rule out the possibility that 26S proteasome undergo very fast dissociation and re-association during translocation through the NPC. To rule out the possibility and show that the holo-complex can enter the NPC, we constructed a strain in which the RP and CP particles were fused: specifically, the CP subunit Pre6 (α4) was genetically fused to the RP subunit Rpt1 or Rpt2 ( Fig. 6a ). The RP-CP–fused strains exhibited wild-type growth even in the presence of oxidative stress ( Fig. 6b ). Because these subunits are essential, the genetic studies suggested that the fusion proteins were functional. Protein bands corresponding to the Rpt1–Pre6 and Rpt2–Pre6 fusion proteins could be detected in the corresponding lysates and in affinity-purified RP-CP–fused proteasomes ( Fig. 6c ; Supplementary Fig. 7 ). The RP–CP proteasome could be purified as the holo-complex even in the absence of ATP ( Fig. 6c , right panel), suggesting that almost all proteasomes contained stoichiometric amounts of the fusion proteins. These observations support the CP template assembly model of the RP [39] . Furthermore, structural analysis by cryo-electron microscopy revealed that the Pre6-Rpt2–fused proteasome was almost indistinguishable from the wild-type proteasome ( Fig. 6d ). Thus, we concluded that the RP-CP–fused proteasomes were functional both in vivo and in vitro . 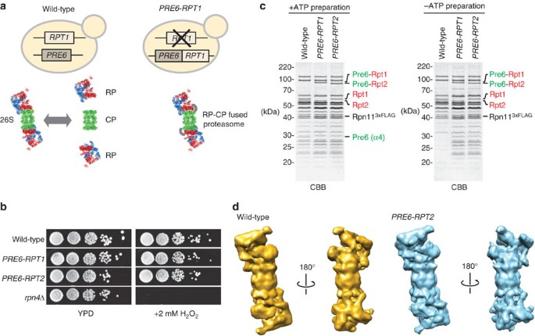Figure 6: Construction of genetically stabilized proteasomes. (a) Construction of the RP-CP–fused proteasome strain. To stabilize the RP–CP interactionin vivo, cells expressing Pre6-Rpt1 or Pre6-Rpt2 fusion protein were generated. (b) The RP-CP–fused cells exhibited wild-type growth. Wild-type (W303-1A), Pre6-Rpt1–fused (YYS961), Pre6-Rpt2–fused (YYS972) andrpn4Δ(YAT1894) cells were spotted onto YPD plates containing 0 or 2 mM H2O2, and then incubated at 25 °C. (c) SDS–polyacrylamide gel electrophoresis (SDS–PAGE) analysis of RP-CP–fused proteasomes. Proteasomes from wild-type (YYS40), Pre6-Rpt1–fused (YYS961) or Pre6-Rpt2–fused (YYS972) cells were affinity-purified using the 3 × FLAG tag in the presence (left) or absence of ATP (right). The proteasomes were subjected to SDS–PAGE followed by coomassie brilliant blue (CBB) staining. Protein bands corresponding to Rpt1, Rpt2, Pre6, Rpn113 × FLAG, Pre6-Rpt1, Pre6-Rpt2, and CP subunits are indicated. A full scan of the gel is provided inSupplementary Fig. 8. (d) Three-dimensional structure of the RP-CP–fused proteasome. Two different views of the cryo-EM maps are represented. The resolution of the wild-type structure is 27 Å, and that of the RP–CP-fused structure is 25 Å. Figure 6: Construction of genetically stabilized proteasomes. ( a ) Construction of the RP-CP–fused proteasome strain. To stabilize the RP–CP interaction in vivo , cells expressing Pre6-Rpt1 or Pre6-Rpt2 fusion protein were generated. ( b ) The RP-CP–fused cells exhibited wild-type growth. Wild-type (W303-1A), Pre6-Rpt1–fused (YYS961), Pre6-Rpt2–fused (YYS972) and rpn4Δ (YAT1894) cells were spotted onto YPD plates containing 0 or 2 mM H 2 O 2 , and then incubated at 25 °C. ( c ) SDS–polyacrylamide gel electrophoresis (SDS–PAGE) analysis of RP-CP–fused proteasomes. Proteasomes from wild-type (YYS40), Pre6-Rpt1–fused (YYS961) or Pre6-Rpt2–fused (YYS972) cells were affinity-purified using the 3 × FLAG tag in the presence (left) or absence of ATP (right). The proteasomes were subjected to SDS–PAGE followed by coomassie brilliant blue (CBB) staining. Protein bands corresponding to Rpt1, Rpt2, Pre6, Rpn11 3 × FLAG , Pre6-Rpt1, Pre6-Rpt2, and CP subunits are indicated. A full scan of the gel is provided in Supplementary Fig. 8 . ( d ) Three-dimensional structure of the RP-CP–fused proteasome. Two different views of the cryo-EM maps are represented. The resolution of the wild-type structure is 27 Å, and that of the RP–CP-fused structure is 25 Å. Full size image Using these strains, we analysed the subcellular distribution of the RP-CP–fused proteasome. As shown in Fig. 7a , proteasome subunits were distributed normally in the nucleus. Importantly, the diffusion properties of the proteasomes measured by FCS were indistinguishable between RP-CP–fused and wild-type cells ( Supplementary Fig. 7c ). Nevertheless, it remained possible that the RP-CP–fused proteasomes assembled in the nucleus. Therefore, we performed nuclear import assays on these proteasomes. In quiescent cells, proteasomes form cytoplasmic granule structures called proteasome storage granules (PSGs) [34] . On addition of fresh medium, PSGs rapidly disappear, and proteasomes re-enter the nucleus within a few minutes [34] . By exploiting this phenomenon, we investigated whether the RP-CP–fused proteasomes could re-enter the nucleus. Because of the low efficiency of PSG formation in our W303 background cells, we used respiration-deficient cells in which intracellular pH rapidly declines on carbon depletion, resulting in efficient formation of PSGs (to be published). Both wild-type and the PRE6-RPT1 –fused cells formed PSGs after 48 h of culture. Strikingly, on the addition of fresh medium, PSGs in both strains rapidly disappeared, and the proteasomes mobilized into the nucleus with the same kinetics ( Fig. 7b ). Thus, RP-CP–fused proteasomes entered the nucleus through the NPC, indicating that dissociation into RP and CP is not required for nuclear import of the assembled proteasome. Taken together, these results suggest that the 26S proteasome can enter the nucleus as the holoenzyme. 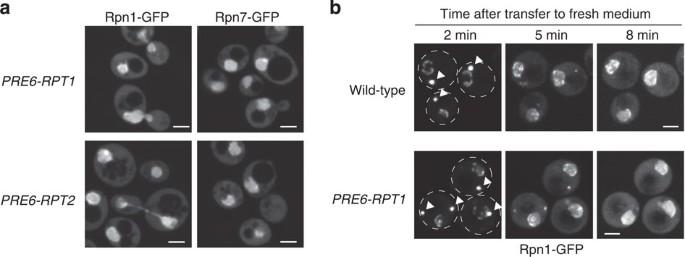Figure 7: Nuclear distribution of genetically stabilized proteasomes. (a) Subcellular distributions of RP-CP–fused proteasomes. Wild-type and RP-CP–fused cells expressing Rpn1-GFP or Rpn7-GFP (YYS1437, YYS1438, YYS1457, YYS1459, YYS1497 and YYS1498) were imaged by confocal microscopy. Scale bars, 2 μm. (b) Assay for nuclear re-import of proteasomes. Wild-type orPRE6-RPT1cells expressing Rpn1-GFP (YYS2117 and YYS2119) were cultured for 2 days to form PSGs. Immediately after transfer to fresh medium, the cells were mounted on glass slides and imaged by confocal microscopy at the indicated time points. PSGs are indicated by arrowheads. Scale bars, 2 μm. Figure 7: Nuclear distribution of genetically stabilized proteasomes. ( a ) Subcellular distributions of RP-CP–fused proteasomes. Wild-type and RP-CP–fused cells expressing Rpn1-GFP or Rpn7-GFP (YYS1437, YYS1438, YYS1457, YYS1459, YYS1497 and YYS1498) were imaged by confocal microscopy. Scale bars, 2 μm. ( b ) Assay for nuclear re-import of proteasomes. Wild-type or PRE6-RPT1 cells expressing Rpn1-GFP (YYS2117 and YYS2119) were cultured for 2 days to form PSGs. Immediately after transfer to fresh medium, the cells were mounted on glass slides and imaged by confocal microscopy at the indicated time points. PSGs are indicated by arrowheads. Scale bars, 2 μm. Full size image In this study, we determined the local concentrations of the proteasome in living yeast cells, and characterized the formation of the proteasome complex, using a quantitative imaging method. Previous studies have demonstrated that the base, base-like complex, and RP function in transcription, independent of the proteolytic function of the proteasome, implying that the proteasome subcomplexes may have specific roles in cells [43] , [44] , [45] . However, our results suggest that the 26S proteasome is a very stable complex, and that free base, RP, and subunits are not present at detectable levels anywhere in the cell, at least under normal culture conditions. In line with our findings, a recent study showed that the transcriptionally relevant form is the canonical 26S proteasome [46] . In a widely accepted model, the precursors of both RP and CP are translocated independently into the nucleus, where they are assembled into the 26S proteasome [19] , [20] , [21] . In contrast to this canonical pathway, our results obtained by FCS/FCCS analysis of the importin mutant and cells expressing genetically stabilized proteasomes ( Fig. 5 ; Supplementary Fig. 7 ) suggest that the 26S proteasome is assembled in the cytoplasm. Because we could not detect proteasome intermediates by FCS, even in the importin mutant, we cannot rule out the possibility of the canonical pathway. Clearly, further studies are needed to clarify which pathway predominates within cells. Regardless, our results strongly suggest that the nuclear import of the precursors is not essential for proteasome assembly ( Fig. 5 ; Supplementary Fig. 6 ). Furthermore, the results of nuclear import assays performed on RP-CP–fused proteasomes suggest that the 26S holoenzyme can translocate through the NPC ( Fig. 7 ). Because the dimensions of the 26S proteasome are 20 nm × 45 nm, we speculate that the proteasome could be transported along its longitudinal axis through the 39-nm NPC channel [25] . The direction and orientation of translocation might be governed by Sts1, an NLS-containing protein that binds the lid subunit Rpn11 (ref. 22 ). In summary, we have demonstrated a method for quantitative imaging analysis that enables direct observation of proteasome dynamics in living yeast cells in which all component proteins expressed at their endogenous levels. We unambiguously determined the local concentrations of the proteasome in distinct subcellular compartments, and also characterized the process of proteasome complex formation. Our live-cell paradigm avoids the potential artifacts of classical biochemical studies of the 26S proteasome, which is a labile complex in vitro . The 26S proteasome is an attractive target for pharmaceutical development [47] , and the proteasome dynamics revealed by ‘ in vivo biochemistry’ provide a new perspective that should facilitate the development of next-generation proteasome inhibitors. Yeast strains and media Strains used in this study are listed in Supplementary Table 1 . Standard protocols were used for yeast manipulation [48] . The proteasome subunits RPN1 , RPN7 and PRE6 were chromosomally tagged with yeast enhanced green fluorescent protein (GFP) or monomeric Cherry fluorescent protein (mCherry), as described previously [21] , [40] , [49] . Genetically stabilized 26S proteasomes in which the CP subunit PRE6 /α4 was fused to the RP subunit RPT1 or RPT2 were constructed as follows. The 5′-truncated PRE6 open reading frame (ORF) (+304 to +762, Not I- Bam HI) was inserted into the Not I- Bam HI site of the yeast-integrating vector pRS306. Next, the RPT1 ORF with its transcriptional terminator (+1 to +1,753, Bam HI- Sal I) or the RPT2 ORF with its terminator (+1 to +1,633, Bam HI- Xho I) was inserted into the Bam HI- Xho I site of pRS306- 5′Δpre6 . The resulting plasmids, pOKA511, pRS306- 5′Δpre6-RPT1 and pOKA512, pRS306- 5′Δpre6-RPT2 , were linearized at the Sal I site within PRE6 and transformed into RPT1/rpt1Δ::LEU2 and RPT2 / rpt2 Δ:: HIS3 , respectively. Ura + transformants were sporulated, and tetrads were dissected. Because RPT1 is an essential gene, Ura − Leu + spores did not germinate. However, we could obtain Ura + Leu + cells, indicating that the PRE6-RPT1 fusion gene complements the RPT1 deletion. Likewise, Ura − His + spores did not germinate, whereas Ura + His + cells could be obtained, indicating that the PRE6-RPT2 fusion gene complements the RPT2 deletion. To generate ρ 0 mutants, cells were cultured in YPD containing 10 μg ml −1 ethidium bromide for 24 h, and diluted cells were streaked onto YPD plates; the resultant colonies were then screened for inability to grow on YPGly plates [50] . Fluorescence correlation spectroscopy Yeast cells chromosomally expressing GFP- and/or mCherry-tagged proteins were grown in SC medium (0.67% yeast nitrogen base without amino acids, 0.5% casamino acids, 2% glucose, 20 mg/l tryptophan, 20 mg/l uracil, 400 mg/l adenine, and 10 mM phosphate buffer, pH 7.5) at 25 °C to logarithmic phase, and then the cultures were shifted to 37 °C for the indicated times. The cells were mounted on a glass-bottom dish (MatTek Corporation). FCS and FCCS measurements were all performed at 25 °C with a ConfoCor2 (Carl Zeiss) microscope, as described [31] , [51] , [52] , [53] . The ConfoCor2 consisted of a CW Ar + and He–Ne lasers, a water-immersion objective (C-Apochromat, 40 × , 1.2 numerical aperture; Carl Zeiss), and two channels of avalanche photodiodes (SPCM-200-PQ; EG&G). GFP was excited with the 488-nm laser line, and RFP with the 543-nm laser line, with the minimal total power that yielded a sufficient signal-to-noise ratio. The confocal pinhole diameter was adjusted to 70 μm for 488 nm and 78 μm for 543 nm. The emission signals were split by a dichroic mirror (570-nm beam splitter) and detected at 505–530 nm in the green channel (for GFP) and 600–650 nm in the red channel (for RFP). Simultaneous excitation of GFP- and mCherry/RFP-tagged proteins was carefully carried out at minimal and optimal excitation powers, chosen to obtain sufficiently high signal-to-noise ratios for analysis of diffusion times while preventing artifacts such as saturation, blinking and photobleaching that might affect the results of such analyses. Because cell and nuclear sizes differ significantly between yeast mother and daughter cells, our FCS and FCCS measurements were carried out on mother cells of similar size throughout the study. However, it should be noted that the FCS/FCCS results did not differ substantially between large mother cells and small daughter cells (data not shown). Data were analysed using the ConfoCor2 software, as described in our previous study. Briefly, the fluorescence auto-correlation functions of the red and green channels, G r ( τ ) and G g ( τ ), and the fluorescence cross-correlation function, G c ( τ ), were calculated from where τ denotes the time delay; I i the fluorescence intensity of the red channel ( i= r) or green channel ( i= g); and G r ( τ ), G g ( τ ), and G c ( τ ) denote the red ( i=j=x= r) and green ( i=j=x= g) auto-correlation functions and the cross-correlation function ( i= r , j= g , x= c), respectively. The acquired G x ( τ ) values were fitted using a one-, two- or three-component model: where F i and τ ı are the fraction and diffusion time of component I , respectively; N is the average number of fluorescent particles in the excitation-detection volume defined by the radius w 0 and the length 2 z 0 ; and s is the structure parameter representing the ratio s=z 0 /w 0 . The structure parameter was calibrated using Rhodamine-6G (Rh6G) standard solution at room temperature. The relationship between absolute concentration and calculated N was calibrated using a known concentration of Rh6G or recombinant mGFP solution. The effect of photobleaching on evaluation of concentration was determined according to a previous study [31] . Fluorescence correlation functions (FCFs) in live cells were measured sequentially 5–10 times with duration of 10 s to minimize the photobleaching effect, because gradual photobleaching by cellular depletion of GFP (RFP) affected diffusion analysis of FCFs obtained from measurements of longer duration ( Supplementary Fig. 1 ). The diffusion time of component i , τ i , is related to the translational diffusion coefficient D of component i by The diffusion of a spherical molecule is related to various physical parameters by the Stokes–Einstein equation as follows. where T is the absolute temperature, r i is the hydrodynamic radius of the spherical molecule, η is the fluid-phase viscosity of the solvent, and κ B is the Boltzmann constant. The diffusion coefficient of GFP-tagged proteins in a solution sample with 1 cP viscosity was evaluated using the known diffusion coefficients (apparent molecular weights) of the Rh6G standard and the recombinant mGFP solutions: respectively, 280 and 78 μm 2 s −1 . For live cells, the diffusion coefficient (apparent molecular weight) of GFP-tagged proteins was evaluated using GFP (or mCherry) expressed in yeast cells. Data containing severe photobleaching, possibly resulting from a high proportion of immobilized fluorophores, were excluded from the diffusion analysis. For FCCS analysis, the amplitude of the cross-correlation function was normalized to the amplitude of the auto-correlation function of mCherry to calculate the relative cross-correlation amplitude ([ G c (0)−1]/[ G r (0)−1]) [28] , [52] , [53] . Interaction amplitude was represented by the relative cross-correlation amplitude corresponding to the fraction of associated molecules ( N c / N g ). All measured FCFs were globally fitted, using the model described above, with the software installed on the ConfoCor 2 system. FCFs of Rh6G, GFP (RFP) and GFP/RFP-tagged molecules in solution were well fitted by a one-component model ( i =1) with or without a triplet term). In living cells, both FCS and FCCS analyses revealed that the mobilities of GFP/mCherry-tagged subunits were well fitted by a two-component model, because the results of analyses using two- and three-component models did not differ significantly. Thus, any third (or higher-order) components were either very weak or otherwise undetectable by these methods. To estimate the diffusion coefficients, FCFs in live cells were fitted by a two-component model ( i =2, D fast and D slow ) with or without a triplet term. Intriguingly, in the two-component analysis, FCFs of GFP- or mCherry-tagged subunits frequently exhibited D fast values with D >10 μm 2 s −1 , much larger than the value calculated from D of Pre6-GFP in solution ( Supplementary Fig. 1 ) and the apparent viscosity of a yeast cell [51] . This fast component with a large D value was barely detected for FCFs of cross-correlation functions, which exclude independent photochemical effects (such as blinking) from the two fluorescent molecules ( Supplementary Fig. 4 ). Therefore, this fast component for GFP- or mCherry-tagged proteins may be an apparent diffusional term, caused by blinking of the probes, even though the time scale of the blinking was different from that reported in a previous study [54] . Such data were excluded from FCS analysis. The details of the simulations of molecular shapes of various proteins from analyses of FCFs were described in our previous studies [31] , [55] , [56] . Fluorescence microscopy Cells grown in SC medium, described above, were mounted on glass slides and observed with a BX52 fluorescence microscope (Olympus) equipped with a UPlanApo 100 × , 1.45 numerical aperture objective (Olympus), a confocal scanner unit CSU22 (Yokogawa) and an ORCA-ER CCD camera (Hamamatsu Photonics), as described previously [21] . Images were processed using the IPLab software (Scanalytics Inc). For proteasome nuclear import assays ( Fig. 7b ), we acquired images at 0.5-μm intervals in the Z focal plane, and then generated maximal projections of Z stacks. Purification of 26S proteasomes and cryo-electron microscopy Intact 26S proteasomes from wild-type yeast and the RP-CP–fused strain were purified using the Rpn11-3 × FLAG tag [57] . The cells cultured in YPD medium were lysed with glass beads in lysis buffer, 50 mM Tris-HCl, pH 7.5, 100 mM NaCl, 10 mM MgCl 2 , 4 mM ATP and 10% glycerol. After removal of the glass beads, extracts were cleared by centrifugation and incubated with anti-FLAG M2 agarose beads (Sigma) for 2 h at 4 °C. Beads were washed three times with the same buffer and the intact 26S proteasomes were eluted with 400 μg ml −1 3XFLAG peptide (Sigma). For enrichment of the double-capped 26S proteasomes, the eluted samples were subjected to a 15–40% sucrose density gradient, subsequently fractionated, and analysed by SDS–polyacrylamide gel electrophoresis. The vitrified samples were imaged using a Tecnai F20 transmission electron microscope [7] . Using XMIPP [58] , we computed 25-Å and 27-Å resolution maps (Fourier–Shell correlation, FSC=0.5) for the wild-type and RP-CP–fused proteasomes from 43,000 and 15,000 single particles, respectively. How to cite this article: Pack, C.-G. et al. Quantitative live-cell imaging reveals spatio-temporal dynamics and cytoplasmic assembly of the 26S proteasome. Nat. Commun. 5:3396 doi: 10.1038/ncomms4396 (2014).